Size-induced enhanced magnetoelectric effect and multiferroicity in chromium oxide nanoclusters The control of the magnetization of a material with an electric field would make the design and the integration of novel electronic devices possible. This explains the renewed interest in multiferroic materials. Progress in this field is currently hampered by the scarcity of the materials available and the smallness of the magnetoelectric effects. Here we present a proof-of-principle experiment showing that engineering large strains through nanoscale size reduction is an efficient route for increasing magnetoelectric coefficients by orders of magnitude. The archetype magnetoelectric material, Cr 2 O 3 , in the form of epitaxial clusters, exhibits an unprecedented 600% change in magnetization magnitude under 1 V. Furthermore, a multiferroic phase, with both magnetic and electric spontaneous polarizations, is found in the clusters, while absent in the bulk. Voltage control of spintronic devices is envisioned through the coexisting permanent magnetic and electric dipole moments in multiferroic magnetoelectric materials [1] , [2] . Related multifunctional devices would greatly benefit from enlarged magnetoelectric coupling, which allows controlling the magnetic properties of devices by applying a bias voltage. Although the magnetoelectric concept dates back to Pierre Curie [3] , in 1894, the number of studied magnetoelectric materials, and a fortiori of magnetoelectric multiferroic materials, is still limited [4] . Furthermore, producing a substantial modification of the magnetization magnitude under electric field is an ongoing challenge. For instance, the archetype magnetoelectric material, Cr 2 O 3 , which is antiferromagnetic and paraelectric, has a magnetoelectric susceptibility of only a few ps m −1 (ref. 5 ). Even under the largest electric fields created across dielectric thin films (10 9 V m −1 ), the change in magnetization would not exceed a few 10 −3 μ B per Cr atom, that is, about 1 emu cm −3 . Strain engineering is envisioned as a possible route for improving magnetoelectric properties [2] with the predicted huge increase of the magnetoelectric coefficients [6] and even the appearance of new multiferroic phases for strained materials [6] , [7] . Small epitaxial structures, which can sustain much larger amounts of stress than the bulk, are thus worth exploring [8] . Here, we investigate highly strained nanometre size chromium oxide particles, imprisoned in a single crystalline dielectric matrix. We provide evidence for the occurrence of spontaneous magnetization and electric polarization in these particles, which not only behave as superparamagnets but also as superparaelectrics. Moreover, we show that their magnetoelectric coefficients are several orders of magnitude larger than the linear terms in bulk Cr 2 O 3 . Their magnetization can be modified by a fraction of μ B per atom, opening the possibility of efficient use of electric field for controlling the magnetization of the material. Fe/MgO:Cr/Fe magnetic tunnel junctions Insight into the magnetoelectric properties of the nanoparticles is obtained through their tunnel magnetoresistance (TMR) signature ( Fig. 1a–c ). For this work, indeed, we fabricated modified Fe/MgO/Fe(001) magnetic tunnel junction (MTJ) stacks [9] by interrupting the growth of the 5- or 5.5-nm thick MgO insulating layer after 2.5 nm to allow the deposition of a small amount of chromium. The epitaxial growth of chromium on a smooth MgO(001) surface follows the Volmer–Weber mode [10] , which results in the formation of nanometric flat clusters, with narrow size distribution ( Fig. 2 ). Following indications of partial oxidation of chromium at the interface with MgO (ref. 11 ), we annealed the stack after growth completion (Methods) in order to achieve full oxidation of the clusters embedded in MgO. For a nominal chromium thickness t Cr =0.5 nm, the resulting particles are typically 2 nm thick and 6 nm wide ( Fig. 1d,e ). 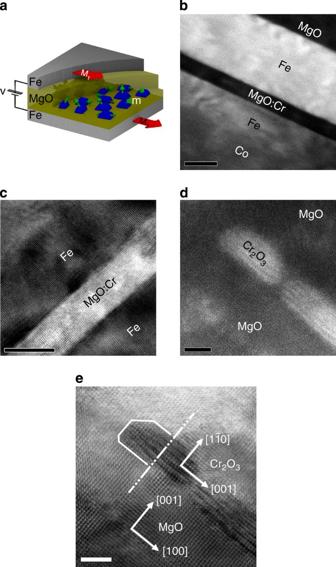Figure 1: Chromium oxide clusters embedded in a MgO tunnel barrier. (a) Schematic of the Fe/MgO:Cr/Fe magnetic tunnel junction devices.M1andM2denote the magnetization vectors of the ferromagnetic electrodes, andmthat of the superparamagnetic granules inside the tunnel barrier. (b,c) Cross-sectional scanning TEM micrographs of a MTJ stack with a nominal Cr thickness of 0.4 nm showing that the inclusion of Cr in the MgO barrier still results in a smooth upper MgO/Fe interface (dark field image, (b) and preserves the epitaxial growth (bright field image,c). (d,e) Cross-sectional views of a 5.5-nm wide, 2-nm thick chromium oxide cluster in a [MgO(3 nm)/Cr(0.5 nm)]10stack. In the high angle annular dark field (Z-contrast) image (d), the Cr2O3cluster appears as brighter in the darker MgO matrix. From the bright field image with atomic resolution (e), one may determine the orientational relationship between bcc MgO and hexagonal Cr2O3: Cr2O3[001]|MgO[100] and Cr2O3[1ī0]|MgO[001] (see Methods). Scale bars, 10 nm (b,c) and 2 nm (d,e). Figure 1: Chromium oxide clusters embedded in a MgO tunnel barrier. ( a ) Schematic of the Fe/MgO:Cr/Fe magnetic tunnel junction devices. M 1 and M 2 denote the magnetization vectors of the ferromagnetic electrodes, and m that of the superparamagnetic granules inside the tunnel barrier. ( b , c ) Cross-sectional scanning TEM micrographs of a MTJ stack with a nominal Cr thickness of 0.4 nm showing that the inclusion of Cr in the MgO barrier still results in a smooth upper MgO/Fe interface (dark field image, ( b ) and preserves the epitaxial growth (bright field image, c ). ( d , e ) Cross-sectional views of a 5.5-nm wide, 2-nm thick chromium oxide cluster in a [MgO(3 nm)/Cr(0.5 nm)] 10 stack. In the high angle annular dark field (Z-contrast) image ( d ), the Cr 2 O 3 cluster appears as brighter in the darker MgO matrix. From the bright field image with atomic resolution ( e ), one may determine the orientational relationship between bcc MgO and hexagonal Cr 2 O 3 : Cr 2 O 3 [001]|MgO[100] and Cr 2 O 3 [1ī0]|MgO[001] (see Methods). Scale bars, 10 nm ( b , c ) and 2 nm ( d , e ). 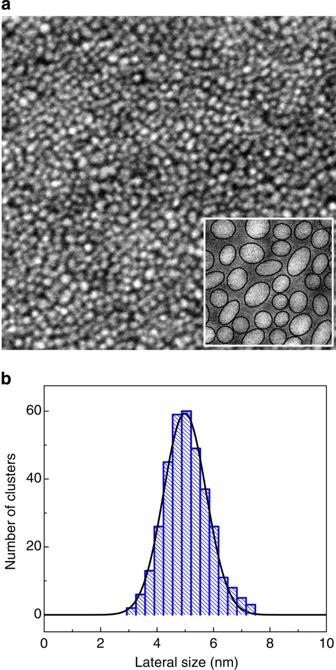Figure 2:Chromium nanoclusters on MgO. (a) 200 × 200 nm2scanning electron microscopy image of the clusters formed on the lower MgO tunnel barrier (tCr=0.5 nm) before deposition of the upper barrier and annealing. The inset in the lower right corner is an illustration of the treatment performed with the ImageJ software (Methods), in which the clusters are supposed to have ellipsoidal shape. (b) Statistical distribution of the cluster size (square root of surface area) as obtained from an analysis of 460 nanoobjects. The distribution is a gaussian peaked at 5.0 nm, with a full width at half-maximum of 1.5 nm. Full size image Figure 2: Chromium nanoclusters on MgO . ( a ) 200 × 200 nm 2 scanning electron microscopy image of the clusters formed on the lower MgO tunnel barrier ( t Cr =0.5 nm) before deposition of the upper barrier and annealing. The inset in the lower right corner is an illustration of the treatment performed with the ImageJ software (Methods), in which the clusters are supposed to have ellipsoidal shape. ( b ) Statistical distribution of the cluster size (square root of surface area) as obtained from an analysis of 460 nanoobjects. The distribution is a gaussian peaked at 5.0 nm, with a full width at half-maximum of 1.5 nm. Full size image Their chemical, structural and magnetic properties were studied by X-ray absorption spectroscopy (XAS) and X-ray magnetic circular dichroism (XMCD). Absorption measurements at the L 2,3 edges of Cr ( Fig. 3a ) show no significant contribution of residual metallic chromium. They indicate that around 90% of Cr atoms are in a +3 oxidation state and reside in an oxygen octahedral environment alike in bulk α-Cr 2 O 3 . Moreover, the largest part (80%) of the XMCD signal ( Fig. 3b ) can be reproduced using the reference spectrum of Cr 3+ ions in ruby α-Al 2 O 3 :Cr 3+ (ref. 12 ), which has the same corundum structure as α-Cr 2 O 3 . Since bulk Cr 2 O 3 is an antiferromagnet, the sizable XMCD signal recorded, proving the existence of a finite magnetization M , should primarily result from spin canting in the Cr 2 O 3 particles. As for the small fraction of atoms in a different environment, it is believed to be located at the boundaries of the clusters. Its contribution to absorption could be crudely reproduced using a reference XAS spectrum of CrO 2 (ref. 13 ). This interfacial phase also contributes to the dichroic signal (20%). This is consistent with a number of previous works reporting imperfect antiferromagnetic compensation of spins at the surface of Cr 2 O 3 nanoparticles (see, for example, ref. 14 ), and with the discovery of a roughness-insensitive magnetization at the surface of bulk Cr 2 O 3 (ref. 15 ). 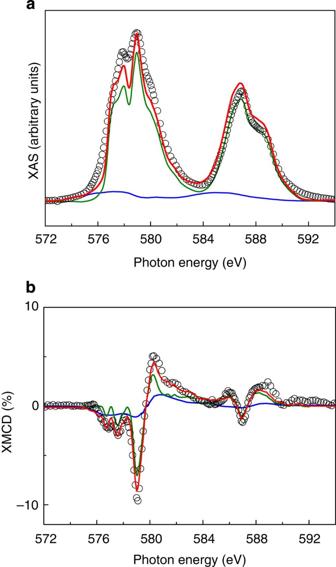Figure 3:Oxidized Cr nanoclusters. (a) Isotropic X-ray absorption spectrum at the CrL2,3edges of an MgO:Cr/Fe/MgO(001) sample with nominal Cr thickness 0.4 nm (symbols). Data were taken at 2 K. The fit (red line) was obtained assuming 93% of Cr atoms in the corundum Cr2O3structure (green line) and 7% in that of CrO2(blue line). (b) XMCD signal on the same sample as ina. The difference in absorption between left and right circularly polarized lights is normalized to the maximum isotropic absorption at 578.9 eV. Chromium atoms in the Cr2O3environment contribute 80% of the integrated signal (same color convention as ina). Figure 3: Oxidized Cr nanoclusters . ( a ) Isotropic X-ray absorption spectrum at the Cr L 2,3 edges of an MgO:Cr/Fe/MgO(001) sample with nominal Cr thickness 0.4 nm (symbols). Data were taken at 2 K. The fit (red line) was obtained assuming 93% of Cr atoms in the corundum Cr 2 O 3 structure (green line) and 7% in that of CrO 2 (blue line). ( b ) XMCD signal on the same sample as in a . The difference in absorption between left and right circularly polarized lights is normalized to the maximum isotropic absorption at 578.9 eV. Chromium atoms in the Cr 2 O 3 environment contribute 80% of the integrated signal (same color convention as in a ). Full size image Determination of the clusters magnetic moment through TMR Tunnel magnetoresistance properties of the Fe/MgO:Cr/Fe devices, very different in shape and amplitude from those of reference Fe/MgO/Fe(001) MTJs (see ref. 9 and Supplementary Fig. 1c ), confirm that the oxidized Cr clusters carry a finite spontaneous magnetic moment ( Fig. 4a ). Indeed, all of the features of the resistance ( R ) versus applied magnetic field ( H ) curves, and especially the characteristic anhysteretic variation of R at large H , can be explained within a model of tunnelling between the ferromagnetic Fe electrodes through superparamagnetic entities [16] . In Supplementary Note 1 , we detail the model and its adequacy for fitting the R ( H ) data and we show that the smallness of the observed TMR effect implies that the conclusions below do not depend on the nature of the tunnelling mechanism (sequential or correlated) effectively involved. 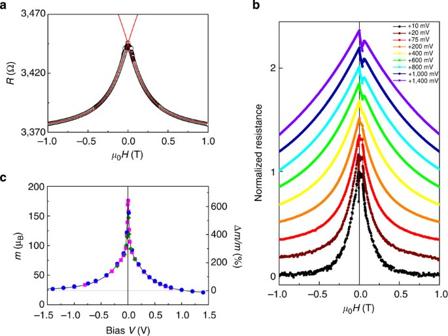Figure 4:Tunnel magnetoresistance effects through the chromium oxide clusters. The data shown are for a device with a nominal Cr thickness of 0.3 nm. (a) TypicalR(H) curve at 6 K under a bias voltageV=130 mV (symbols) and fit to the experimental data assuming sequential tunneling through superparamagnetic clusters with magnetic momentm=78 μB(line). (b) NormalizedR(H) curves for increasing bias voltages between 10 mV (black) and 1.4 V (violet). For the sake of clarity, curves are shifted and only the increasing field branch is shown. (c) Variation of the magnetic moment of the clustersmwith the applied voltageVas deduced fromR(H) curves at 6 K. Data for four different devices of the same sample are shown with different symbols. The lines are guides to the eyes. Figure 4: Tunnel magnetoresistance effects through the chromium oxide clusters . The data shown are for a device with a nominal Cr thickness of 0.3 nm. ( a ) Typical R ( H ) curve at 6 K under a bias voltage V =130 mV (symbols) and fit to the experimental data assuming sequential tunneling through superparamagnetic clusters with magnetic moment m =78 μ B (line). ( b ) Normalized R ( H ) curves for increasing bias voltages between 10 mV (black) and 1.4 V (violet). For the sake of clarity, curves are shifted and only the increasing field branch is shown. ( c ) Variation of the magnetic moment of the clusters m with the applied voltage V as deduced from R ( H ) curves at 6 K. Data for four different devices of the same sample are shown with different symbols. The lines are guides to the eyes. Full size image Because of the superparamagnetic behaviour of the clusters assembly, TMR probes the spatial and thermal average of cos θ , where θ is the angle of the cluster magnetic moment m ( Fig. 1a ) with respect to the applied magnetic field direction. The R ( H ) curve follows , where μ 0 is the magnetic permeability of vacuum, k B is the Boltzmann constant, and is the Langevin function. Hence, at fixed temperature T , the aspect of the TMR curve reflects the magnitude of the magnetic moment of the individual nanoparticles, m , which can be readily extracted from the data ( Fig. 4a and Supplementary Note 1 ). For 5-nm wide, 2-nm thick clusters and small bias voltage, m reaches typically 130 μ B at 6 K, that is about 0.08 μ B per Cr atom (of the order of 30 emu cm −3 ). This value, much smaller than the magnetic moment of Cr 3+ ions in bulk Cr 2 O 3 (2.48 μ B ) (ref. 17 ), confirms that the finite magnetization of the chromium oxide clusters originates from spin canting (weak ferromagnetism). Temperature dependence of the R(H) curves A characteristic feature of superparamagnetic assemblies is that their magnetization M scales as H / T . This results from the fact that M follows a Langevin function with argument ( μ 0 mH )/( k B T ) and requires that the magnetic dipole moment of each individual nanomagnet be temperature independent. 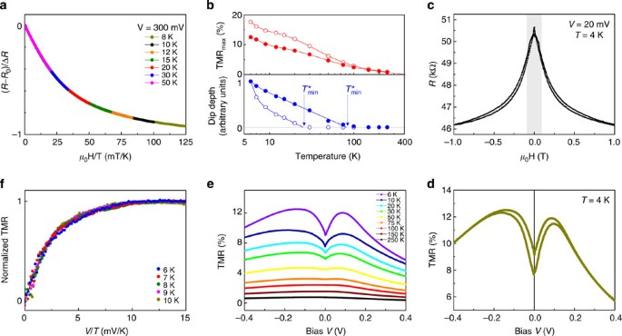Figure 5: Thermal behaviour of the superparamagnetic/superparaelectric phase. The data shown are from three different samples withtCr=0.19 nm (b),tCr=0.40 nm (a,f) andtCr=0.74 nm (b–e). The two extreme values correspond, respectively, to the smallest and largest clusters investigated in the present work. (a)R(H) data taken at different temperaturesTon decreasing the magnetic field from 1 T to 0 T plotted againstH/T. The data have been normalized to account for the temperature dependence of the magnetoresistance (ΔR) and zero magnetic field resistance (R0) of the device. (b) Temperature variations of the maximum TMR ratio (top) and relative depth of the low-bias dip (bottom) for the largest (solid symbols) and smallest clusters (open symbols). (c,d) HystereticR(H) (c) andTMR(V) (d) curves obtained at 4 K for the largest clusters. (e)TMR(V) curves at various temperatures between 6 K and 250 K (largest clusters). (f)TMR(V) data at different temperatures plotted againstV/T. The raw data have been normalized to eliminate the temperature dependence of the depth of the low-bias dip. Figure 5a shows that the R ( H ) data recorded on Fe/MgO:Cr/Fe MTJs closely obey such a scaling law. Figure 5: Thermal behaviour of the superparamagnetic/superparaelectric phase. The data shown are from three different samples with t Cr =0.19 nm ( b ), t Cr =0.40 nm ( a , f ) and t Cr =0.74 nm ( b – e ). The two extreme values correspond, respectively, to the smallest and largest clusters investigated in the present work. ( a ) R ( H ) data taken at different temperatures T on decreasing the magnetic field from 1 T to 0 T plotted against H / T . The data have been normalized to account for the temperature dependence of the magnetoresistance (Δ R ) and zero magnetic field resistance ( R 0 ) of the device. ( b ) Temperature variations of the maximum TMR ratio (top) and relative depth of the low-bias dip (bottom) for the largest (solid symbols) and smallest clusters (open symbols). ( c , d ) Hysteretic R ( H ) ( c ) and TMR ( V ) ( d ) curves obtained at 4 K for the largest clusters. ( e ) TMR ( V ) curves at various temperatures between 6 K and 250 K (largest clusters). ( f ) TMR ( V ) data at different temperatures plotted against V / T . The raw data have been normalized to eliminate the temperature dependence of the depth of the low-bias dip. Full size image The superparamagnetic state classically occurs within a limited temperature range. It evolves at lower temperatures towards a blocked state (measurement time shorter than the characteristic time between two flips of the magnetization) and makes a phase transition to the high temperature paramagnetic state at the magnetic Curie point T C m . Here, the persistence of a still sizable TMR at 250 K ( Fig. 5b,e ) indicates that the clusters likely remain magnetically ordered up to nearly room temperature. On the other hand, signs of blocking of the magnetic dipole moments are observed upon lowering of the temperature down to 4 K. For the largest clusters investigated in the present work (mean diameter ‹ d ›=7.3 nm), this occurs just below 6 K. The signature of this blocking takes the form of a hysteresis in the R ( H ) loop ( Fig. 5c ) at magnetic fields much larger than the saturation field of the Fe electrodes ( Supplementary Fig. 1b,c ). Very much like the magnetization isotherms of assemblies of monodispersive magnetic nanocrystals [18] , the resistance loop then contains both reversible and irreversible contributions. Electric field dependence of the magnetic moment The aspect of the R ( H ) curve strongly depends on the applied bias voltage V ( Fig. 4b ). This reveals that the cluster magnetic moment is highly sensitive to the electric field E . We find that m strongly decreases with increasing voltage ( Fig. 4c ), the relative change reaching 600% between 5 mV and 1 V. We note that the variation of m with V is fully reproducible from one MTJ to another if the devices are fabricated under the same conditions. At this point, one needs to rule out the possibility that the decrease of m with V be related to the dispersion in the cluster size: conduction through the smallest nanoparticles, a priori those with the smallest magnetic moments, could be hindered by Coulomb blockade at small bias voltage. This would give rise to an artificially enhanced average magnetic moment as V approaches zero [19] . A couple of strong arguments may be put forward against this scenario. First, the magnetic moment carried by the Cr 2 O 3 clusters varies with size in a counterintuitive and non-monotonous manner ( Fig. 6a ) so that the opposite behaviour, (that is, an increase of m with V ), would rather be observed, should Coulomb blockade govern the changes of m (see Supplementary Fig. 2 and Supplementary Note 2 ). Second, large changes of m with V still occur when the potential energy eV is much larger than the charging energy of the clusters , where is their estimated capacitance ( Supplementary Fig. 2b ). We therefore ascribe our observations to a large intrinsic magnetoelectric effect in the Cr 2 O 3 nanoparticles. 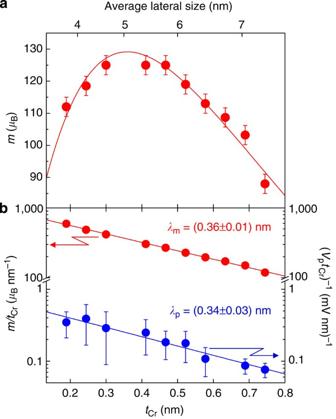Figure 6:Influence of the size of the chromium oxide clusters on the ferroic order parameters. (a) Average magnetic moment of the clustersm, at 6 K and under −10 mV bias voltage, as a function of the nominal thickness of chromium depositedtCr(bottom scale) or average cluster size (top scale). The line is a fit according tom(tCr)=m0exp(−tCr/λm)tCr, withm0=966 μBandλm=0.36 nm. (b) Semi-logarithmic plot ofm/tCr(magnetization, red symbols) and (VptCr)−1(electric polarization, blue symbols) versustCr, and linear fits (lines) to the experimental data. The error bars are derived from the standard errors of the least-squares fits performed to extractmandVpfromR(H) andTMR(V) data curves. Figure 6: Influence of the size of the chromium oxide clusters on the ferroic order parameters . ( a ) Average magnetic moment of the clusters m , at 6 K and under −10 mV bias voltage, as a function of the nominal thickness of chromium deposited t Cr (bottom scale) or average cluster size (top scale). The line is a fit according to m ( t Cr )= m 0 exp (− t Cr / λ m ) t Cr , with m 0 =966 μ B and λ m =0.36 nm. ( b ) Semi-logarithmic plot of m / t Cr (magnetization, red symbols) and ( V p t Cr ) −1 (electric polarization, blue symbols) versus t Cr , and linear fits (lines) to the experimental data. The error bars are derived from the standard errors of the least-squares fits performed to extract m and V p from R ( H ) and TMR ( V ) data curves. Full size image The strongly nonlinear and almost even variation of m with V ( Fig. 4c ) suggests that quadratic terms in E dominate the magnetoelectric behaviour. This is in agreement with the drastic increase of the quadratic magnetoelectric coefficient predicted in nanoclusters [6] as well as with the poor symmetry compatibility between weak ferromagnetism and linear magnetoelectric effect [20] . Yet, m does not vary as V 2 . In order to evaluate the sensitivity of magnetization to electric field, we define a voltage-dependent effective magnetoelectric coefficient as , where is the average volume of the clusters. Under the assumption that the electric field between the metal electrodes is homogeneous, we find α eff =6.7 ns m −1 at low bias (10 mV, Fig. 4c ). This is three orders of magnitude higher than the maximum linear coefficient reported for bulk Cr 2 O 3 , α=4.17 ps m −1 at 263 K (ref. 5 ). Note that α eff goes down to 29 ps m −1 at 1 V, which is still large compared with bulk. Influence of the clusters size on the magnetization To investigate the influence of the size of the nanoparticles, we grew samples with a gradient in the nominal thickness of chromium such that 0.1 nm< t Cr <0.8 nm. Along the gradient, the height ( h =2 nm) and the density ( σ =2 × 10 4 μm −2 ) of the clusters are nearly constant (ref. 10 and Methods) and, consequently, the in-plane surface area and the volume of the clusters are proportional to t Cr —see Fig. 6 for the correspondence between t Cr and cluster size. Figure 6a shows the variation of m with t Cr as extracted from magnetotransport measurements taken on different MTJs along the gradient. As already mentioned before, m does not increase monotonously with the size of the particles. Instead, it exhibits a broad maximum at nm. According to what precedes, m / t Cr is proportional to the magnetic moment per Cr atom, that is, to magnetization. As illustrated in Fig. 6b , this ratio diminishes exponentially as the size of the nanoparticles increases. The same behaviour with a characteristic decay constant of λ m =(0.36±0.01) nm is found whatever the applied voltage and the temperature. In the epitaxial growth of quantum dots, following either the Volmer–Weber or the Stranski–Krastanov modes, the introduction of dislocations [21] and the elastic relaxation at the dot edges [22] often yield an exponential relaxation of stress with increasing layer thickness. The epitaxial relationship between the Cr 2 O 3 inclusions and the surrounding MgO matrix implies nominal in-plane compressive strains of −7% along the c axis of the corundum structure, and of −18% perpendicular to it (Methods). In epitaxial clusters, such a large lattice mismatch usually starts relaxing from the beginning of growth [22] . For t Cr =0.4 nm, photoluminescence spectra ( Fig. 7a ) taken on a large ensemble of nanoparticles are indicative of average compressive stress in excess of 6 GPa and, for t Cr =0.5 nm, observations of six individual clusters by scanning transmission electron microscopy with atomic resolution ( Figs 1e , 7b , Supplementary Table 1 ) reveal an actual strain along c in the range of −3 to −6%, consistent with a partial structural relaxation. On the basis of these considerations, we consider the exponential decay of m / t Cr with t Cr as a strong indication that compressive epitaxial strain is responsible for the finite magnetization of the chromium oxide clusters. This is consistent with recent experimental works [23] , [24] reporting a remnant magnetic moment in granular Cr 2 O 3 arising from magneto-elastic effects. Note that, following the model of Glinchuk et al. [6] , non-zero magneto-elastic coefficients can explain the drastic enhancement of magnetoelectric properties we observe in strained Cr 2 O 3 clusters. 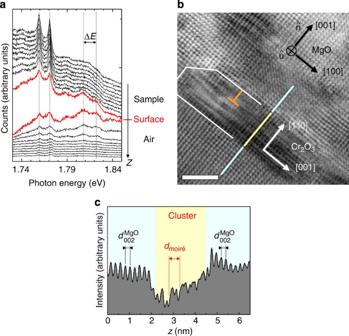Figure 7:Evidence of compressive strain in the chromium oxide clusters. (a) Micro-photoluminescence spectra obtained at different focalisation height on an MgO:Cr/Fe/MgO(001) stack withtCr=0.4 nm. A spectrum was recorded every 0.5 μm, fromz=+5.5 μm above the nominal position of the sample surface (bottom) toz=−4.5 μm below (top). The high energy peaks (1.81–1.82 eV), the intensity of which is the strongest when the laser beam is focused close to the sample surface (thick red lines), are attributed to emission from Cr3+ions in the Cr2O3clusters. The energy difference between these R1and R2lines (ΔE=13 meV) is consistent with an average compressive stress in excess of 6 GPa (Methods). (b) High resolution image of an exceptionally large cluster (10 nm wide, 2.3 nm thick) in an [MgO(3 nm)/Cr(0.5 nm)]10multilayer stack. A dislocation is observed close to its upper surface (orange sign). Scale bar, 2 nm. (c) Intensity profile along the coloured line inb, which is parallel to the normal to the film. Thedmoiré=0.45 nm periodicity of the contrast in the cluster (yellow) region corresponds to parallel moiré fringes formed by the overlapping of (200) MgO planes with spacing =0.215 nm and (300) Cr2O3planes with spacing =0.145 nm, (dmoire)−1=()−1−()−1. Figure 7: Evidence of compressive strain in the chromium oxide clusters . ( a ) Micro-photoluminescence spectra obtained at different focalisation height on an MgO:Cr/Fe/MgO(001) stack with t Cr =0.4 nm. A spectrum was recorded every 0.5 μm, from z =+5.5 μm above the nominal position of the sample surface (bottom) to z =−4.5 μm below (top). The high energy peaks (1.81–1.82 eV), the intensity of which is the strongest when the laser beam is focused close to the sample surface (thick red lines), are attributed to emission from Cr 3+ ions in the Cr 2 O 3 clusters. The energy difference between these R 1 and R 2 lines (Δ E =13 meV) is consistent with an average compressive stress in excess of 6 GPa (Methods). ( b ) High resolution image of an exceptionally large cluster (10 nm wide, 2.3 nm thick) in an [MgO(3 nm)/Cr(0.5 nm)] 10 multilayer stack. A dislocation is observed close to its upper surface (orange sign). Scale bar, 2 nm. ( c ) Intensity profile along the coloured line in b , which is parallel to the normal to the film. The d moiré =0.45 nm periodicity of the contrast in the cluster (yellow) region corresponds to parallel moiré fringes formed by the overlapping of (200) MgO planes with spacing =0.215 nm and (300) Cr 2 O 3 planes with spacing =0.145 nm, ( d moire ) −1 =() −1 −() −1 . Full size image Voltage dependence of the TMR ratio The voltage dependence of the TMR ratio defined as 1− R ( H =1 T )/ R ( H =0) shows remarkable low-bias features ( Fig. 8 ), up to about 80 K ( Fig. 5b,e ). In addition to the overall bell shape usually seen for Fe/MgO/Fe junctions [9] , we observe for the Fe/MgO:Cr/Fe devices a dip in the (−80 mV,+80 mV) voltage range. Similar features have already been reported by Yang and coworkers [25] for TMR stacks with embedded nanometric clusters made of a CoFe metallic alloy. The authors have attributed the dips to a Kondo effect in the ferromagnetic clusters that opens an additional spin-independent conduction channel at low voltage. Unlike in ref. 25 , we do not observe the increase in conductance near zero bias voltage ( Supplementary Fig. 2c ) indicative of a Kondo resonance [26] . Therefore, we rule out such an explanation here. In the following, we propose an explanation in terms of ferroelectricity. 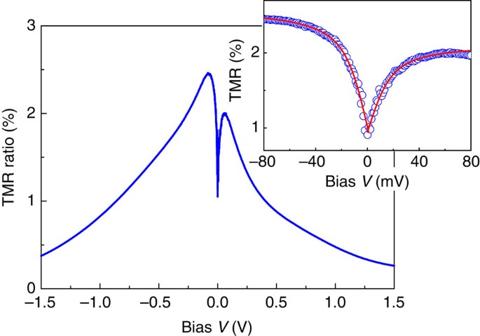Figure 8:Bias dependence of TMR. Variation of the TMR ratio with the applied voltage, at 6 K, for a device withtCr=0.3 nm. The inset shows a zoom in the low voltage range of theTMR(V) curve (symbols) and fits of the experimental data (lines) to the expression, withTMR0=0.99% andVp=7.1 mV. To account for the usual asymmetry of the bias dependence of TMR in Fe/MgO-based magnetic tunnel junctions9, different values ofTMR1were allowed for positive (1.14%) and negative (1.61%) voltages. Figure 8: Bias dependence of TMR . Variation of the TMR ratio with the applied voltage, at 6 K, for a device with t Cr =0.3 nm. The inset shows a zoom in the low voltage range of the TMR ( V ) curve (symbols) and fits of the experimental data (lines) to the expression , with TMR 0 =0.99% and V p =7.1 mV. To account for the usual asymmetry of the bias dependence of TMR in Fe/MgO-based magnetic tunnel junctions [9] , different values of TMR 1 were allowed for positive (1.14%) and negative (1.61%) voltages. Full size image Theoretical works on MTJs with ferroelectric insulating barrier [27] predict that the orientation of the electric polarisation can influence the electron density of states at the ferromagnetic/insulator interfaces and modify the asymmetry between majority and minority electrons. Such modification implies a change in the spin polarisation of the tunnelling electrons and should therefore show up in TMR properties. Consistently, Garcia et al. [28] have observed an abrupt change in TMR on reversal of the polarisation of a BaTiO 3 tunnel barrier. Here no such abrupt change is observed but, in the low-bias range, the TMR curve may be fitted to the equation (see inset in Fig. 8 ), where TMR 0 and TMR 1 are constants, V p is a characteristic voltage value, and is again the Langevin function. We therefore argue that the Cr 2 O 3 clusters are ferroelectrically ordered and that they behave as superparaelectrics. The concept of superparaelectricity was defined many years ago [29] by analogy with superparamagnetism. It should become increasingly relevant in the search of ferroelectricity at the nanoscale [30] and, indeed, a recent work on BaTiO 3 nanocubes also reports a possible signature of this effect [31] . In the superparaelectric state, the permanent electric dipole moments of small enough ferroelectric particles fluctuate in direction because thermal energy exceeds the energy barrier against polarisation rotation. Applying an electric field E to an assembly of such particles orients their electric dipoles preferentially in the direction of E and the resulting total electric polarisation follows a Langevin law. The dip in the TMR ( V ) curve reflects such a behaviour. The way it changes with temperature also ascertains the superparaelectric nature of the Cr oxide clusters. Indeed, in the temperature range where the bell-shaped background TMR signal evolves little in shape, the low-bias part of the TMR ( V ) curves obeys the expected V / T scaling ( Fig. 5f ), which is the pendant of the H / T scaling in superparamagnetism ( Fig. 5a ). Taking the electric field as homogeneous through the entire MgO/Cr 2 O 3 /MgO stack of total thickness d ~6 nm ( E = V / d ), one can evaluate the average electric dipole p of the Cr 2 O 3 clusters from ( V )/( V p )=( pE )/( k B T ). For t Cr =0.3 nm ( Fig. 8 ), we get p =7.4 × 10 −29 C m. The corresponding electric polarization P is of the order of 0.22 μC cm −2 . It is small compared to that of the archetypical material BiFeO 3 (ref. 32 ), but of the same order of magnitude as those of improper ferroelectrics where the spontaneous polarization is a secondary-order parameter induced by lattice distortion [33] , [34] . It is also of the same order of magnitude as the value of 0.585 μC cm −2 calculated by Mostovoy et al. [35] for Cr 2 O 3 in a hypothetical multiferroic state realized by reversing one out of four spins in the rhombohedral unit cell. Such a low polarisation value favours the occurrence of superparaelectricity. First, it makes the electrostatic interactions between clusters weak and thus prevents the formation of a globally ordered state [36] . Second, it implies a low energetic barrier against polarisation rotation, which is an even stronger requirement. This energy barrier scales as P 2 (refs 30 , 36 ) and its size is of the order of the energy W C of a ferroelectric capacitor with volume V : W C =(1)/(2) VP 2 /εε 0 (ref. 30 ), where ε 0 is the permittivity of vacuum. For Cr oxide clusters with dielectric constant (at least), volume V =35 nm 3 , and polarisation P =0.22 μC cm −2 ( t Cr =0.3 nm), W C amounts to 5.4 meV, which is equivalent to 60 K. We note that this is the right order of magnitude for observing superparaelectricity down to temperatures of a few Kelvin. By analogy with superparamagnetism, one expects that the superparaelectric state be preceded by a blocked state at lower temperatures and, indeed, a sign of the blocking of (some of) the electric dipole moments in the form of a hysteresis in the TMR ( V ) data is observed for the largest clusters, below 6 K ( Fig. 5d ). On the high temperature side, the superparaelectric state should be followed by a paraelectric state beyond the electric Curie point . We note that the low-bias dip in the TMR ( V ) curve, which we consider as a signature of the electric ordering, disappears beyond a temperature which increases from for the smallest clusters considered in the present study (mean diameter ‹ d ›=3.7 nm) to for the largest ones (‹ d ›=7.3 nm), see Fig. 5b . However, since TMR is an indirect probe of the ferroelectricity of the clusters, T * should only be considered, at best, as a lower bound for . A strong and final argument for the occurrence of ferroelectric ordering in the clusters is brought by the size dependence of V p . Just as m / t Cr is a measure of the clusters magnetization, ( V p t Cr ) −1 should be a measure of their electric polarization. As seen in Fig. 6b , ( V p t Cr ) −1 also decreases exponentially with increasing t Cr , with a characteristic decay constant λ p =(0.34±0.03) nm very close to that of the magnetization, λ m . There is therefore experimental evidence that the two dipoles, p and m , share a common origin: epitaxial strain drives the value of the magnetic dipole m as well as that of the electric dipole p . The occurrence of a permanent electric polarisation under stress in paraelectric materials with non-zero coupling between lattice and electric order has indeed been predicted [6] , [7] , [37] and observed [8] in other systems. We thus conclude that the Cr 2 O 3 particles exhibit both a (weak) ferromagnetic order and a ferroelectric order. In summary, the ferroic properties of Cr 2 O 3 are drastically changed at the nanoscale. Epitaxial Cr 2 O 3 nanoclusters imprisoned in a single crystalline MgO matrix experience large compressive strain that makes an original superparamagnetic/superparaelectric phase appear. The clusters also exhibit large magnetoelectric effects with effective coefficients in the ns m −1 range, which compare with those obtained in piezoelectric/piezomagnetic nanocomposites [38] . Combined with superparamagnetism, these large effects imply a very strong electric field dependence of the magnetic susceptibly or electro-inductance effect. It can be regarded as the symmetric effect of the intensively studied magneto-capacitance phenomenon [33] and could find important applications outside the field of spintronics, for instance, to build devices with electric field-controlled inductance. Thin film growth and MTJ fabrication The epitaxial (001) oriented heterostructures were grown by molecular beam epitaxy on (001) MgO substrates. The multilayers were deposited at 470 K, and subsequently annealed at 720 K for one hour in ultrahigh vacuum. The final stacking sequence is Pt(2)/Co(15)/Fe(5)/MgO(2.5 or 3)/Cr( t Cr )/MgO(2.5)/Fe(20)/MgO, where thicknesses are given in nm. The top Fe/Co bilayer is the magnetically harder electrode. In some cases, a gradient in Cr thickness was realized by moving progressively a shutter across the sample during deposition. Tunnel junction devices with diameter of 8–30 μm were patterned using standard microfabrication techniques, including UV lithography, Ar ion etching, encapsulation with Si oxide and metal (Al/Au) liftoff to realize the top electrical contact. Scanning electron microscopy observations Scanning electron microscopy was used to observe the Cr clusters formed on the MgO/Fe/MgO(001) surface before being covered with MgO and annealed. An example of micrograph obtained for t Cr =0.5 nm, shortly after deposition, is shown in Fig. 2 , together with the corresponding distribution of cluster lateral size as deduced from an image analysis performed with the ImageJ software. The scattering in the size of the clusters is rather moderate: the diameter distribution is a gaussian peaked at 5.0 nm, with a full width at half-maximum of 1.5 nm. Images taken along a Cr wedge 0.2 nm 0.6 nm indicate that, within 5%, the cluster density remains constant (approximately 2 × 10 4 μm −2 ) as the amount of metal deposited increases, in agreement with previous observations by Koda et al. [10] Magnetotransport experiments Measurements were carried out using a conventional DC 4-wire technique, with the positive reference for voltage taken at the top (Fe/Co) electrode and the external magnetic field applied along the [100] easy direction of magnetization of the bcc Fe layers. The TMR ( V ) curves were obtained by combining current-voltage characteristics measured successively, with external magnetic fields of 1 T and 0 T. No significant difference in the magnetotransport data could be observed whether or not a magnetic field and/or an electric field was applied during cooling of the sample from room temperature down to 6 K. X-ray absorption experiments XAS and XMCD measurements were performed at 2 K on a dedicated MgO:Cr/Fe/MgO(001) sample with t Cr =0.4 nm, using the cryomagnetic endstation available at the DEIMOS beamline of SOLEIL synchrotron. The absorption was measured at the L 2,3 edges of Cr through the total electron yield with a large beam size of about 800 × 800 μm 2 and a low photon flux so as to avoid charging electrically the sample. The presence, below the MgO layer containing the clusters, of a 20-nm thick metal film much thicker than the light penetration depth (a few nanometres) excluded any contribution to the recorded spectra from the Cr 3+ ionic impurities usually present in bulk MgO substrates [39] . The XMCD signal was obtained by combining XAS spectra recorded with left and right circularly polarized lights and applied magnetic fields of +6 T and −6 T. Experimental data were fitted to a linear superposition of reference spectra found in the literature for bulk α-Cr 2 O 3 (XAS) [40] , Cr 3+ ions in ruby α-Al 2 O 3 :Cr 3+ (XMCD) [12] and a thick CrO 2 film (XAS and XMCD) [13] . Scanning transmission electron microscopy observations STEM in cross section was used to characterize the morphology of the MgO tunnel barrier, visualize the embedded clusters and determine their epitaxial relationship and the related lattice mismatch with the matrix material. STEM images show that, despite the inclusion of Cr, the MgO barrier has uniform thickness and smooth interfaces ( Fig. 1b ). The clusters have almost equal height ( h =2 nm) while their lateral dimensions are within the 4–8 nm range for t Cr =0.5 nm. Atomic resolution pictures reveal that crystalline planes are continuous throughout the MgO matrix and the clusters ( Figs 1f , 7b ), meaning that the latter are still epitaxial after being covered and annealed/oxidized. No clear micro-diffraction patterns could be obtained on such clusters. Yet, atomic planes parallel to both the normal to the film and the zone axis ([010] direction of MgO) in Fig. 7b have (0.218±0.002) nm periodicity, which is close to the distance between (006) planes in bulk Cr 2 O 3 , =0.227 nm (here Miller indices for chromium oxide refer to the hexagonal unit cell). Moreover, the distance between atomic planes perpendicular to ((0.145±0.004) nm, Fig. 7c ) matches that between (300) planes in bulk, =0.143 nm. This shows that the c axis of the corundum structure lies in the plane of the layers, parallel to the [100] direction of MgO. Overall, the orientational relationship between the matrix and cluster materials can be summarized as follows: Cr 2 O 3 [001]||MgO[100] and Cr 2 O 3 [1ī0]||MgO[001]. This is fully consistent with i) the epitaxial growth of bcc Cr(001) on MgO(001) with the well-known orientational relationship Cr[100]||MgO[110] and ii) the fact that Cr 2 O 3 formed by oxidation of metallic Cr usually obeys Cr 2 O 3 [001]||Cr[110] (refs 41 , 42 ), and sometimes also Cr 2 O 3 [1ī0]||Cr[001] (ref. 42 ). From the orientational relationship, the lattice mismatch between the matrix and cluster materials can be estimated: 1−/=−7% along the c axis direction, and 1−/=−18% along the in-plane direction that is perpendicular to c . Cr oxide nanoparticles imprisoned in the Mg oxide matrix are then bound to be under strong in-plane biaxial compressive stress. Because of stress relaxation through the introduction of dislocations, such as the one which is visible in Fig. 7b , and deformation at the cluster edges, the actual in-plane strain is, however, reduced. In the cluster of Fig. 7b , the strain along c amounts to −(4±1)%, which, with a Young modulus of 315 GPa (ref. 43 ), corresponds to a large stress of −(13±3) GPa. All the clusters that were observed by STEM showed similar compressive in-plane strains ( Supplementary Table 1 ). Along , the distance between atomic planes is measured with too large an error bar that prevents strain evaluation. Micro-photoluminescence The photoluminescence and Raman spectra of Cr 3+ ions are known to be sensitive to the hydrostatic or biaxial stress in corundum structures [44] , [45] , [46] . More precisely, Nychka et al. [44] and Selcuk et al. [45] showed that the R 1 and R 2 luminescence lines have different piezo-spectroscopic coefficients so that the energy difference between them, Δ E , which is 4 meV in unstressed samples, increases with increasing compressive stress. It was demonstrated experimentally [44] that, up to a biaxial stress of 6 GPa, Δ E is linear in stress and increases by about 0.1 meV per GPa. Above 6 GPa, no systematic measurements were carried out but a nonlinear behaviour is expected [45] . To further ascertain the presence of strain in our chromium oxide clusters, we therefore recorded micro-photoluminescence spectra in a backscattering configuration using a laser beam at 2.33 eV with a Rayleigh length of about 1 μm. To avoid light absorption, we used a dedicated sample ( t Cr =0.4 nm) without top electrode but with a 20 nm bottom Fe electrode acting as a semi-transparent mirror. Spectra recorded at varying focalisation height z of the laser beam ( Fig. 7a ) show two close peaks in the 1.76–1.77 eV energy range, irrespective of z . Since these are also present in the spectra of bare MgO substrates, one can ascertain that they arise from impurities which are systematically present in bulk MgO, with concentrations in the tens of p.p.m. range [39] . The observed peaks coincide quite well with the R-line (1.776 eV) from Cr 3+ ions in octahedral symmetry sites and the N-lines (1.773 and 1.762 eV) associated with Cr 3+ ions in tetragonal symmetry sites [47] . When the beam is focused on the surface ( ), the luminescence spectrum exhibits two extra peaks at higher energy (1.81–1.82 eV), which are interpreted as the R 1 and R 2 emission lines of Cr 3+ ions in the chromium oxide clusters. The energy difference Δ E between them (13 meV) is much larger than in unstrained materials and exceeds the value associated with the 6 GPa maximum stress investigated in refs 44 , 45 . This indicates that an average stress in excess of 6 GPa is present in the clusters, in qualitative agreement with TEM observations. How to cite this article: Halley, D. et al. Size-induced enhanced magnetoelectric effect and multiferroicity in chromium oxide nanoclusters. Nat. Commun. 5:3167 doi: 10.1038/ncomms4167 (2014).